Ancient homology underlies adaptive mimetic diversity across butterflies Convergent evolution provides a rare, natural experiment with which to test the predictability of adaptation at the molecular level. Little is known about the molecular basis of convergence over macro-evolutionary timescales. Here we use a combination of positional cloning, population genomic resequencing, association mapping and developmental data to demonstrate that positionally orthologous nucleotide variants in the upstream region of the same gene, WntA , are responsible for parallel mimetic variation in two butterfly lineages that diverged >65 million years ago. Furthermore, characterization of spatial patterns of WntA expression during development suggests that alternative regulatory mechanisms underlie wing pattern variation in each system. Taken together, our results reveal a strikingly predictable molecular basis for phenotypic convergence over deep evolutionary time. As different organisms evolve similar phenotypes in response to the same selective pressure, is evolution constrained by genetic architecture or, as Mayr [1] famously postulated, do many roads lead to Rome? Phenotypic convergence can arise from molecular convergence at one or more functional levels (that is, mutation, gene, pathway and so on) or by totally independent means. Given the opportunity for widespread functional diversity, a long-standing question in biology is whether evolution is predictable and, if so, under what circumstances? Our knowledge about the molecular basis of convergent evolution comes primarily from examples of convergence among closely related populations or species in response to a shared environment [2] , [3] , [4] , [5] . This work suggests that re-use of genes and pathways is common on short evolutionary timescales [6] , [7] , but there is an expectation that the constraints that promote molecular convergence should erode over evolutionary time, leading to a diversity of functional mechanisms in comparisons among distantly related organisms [1] , [6] , [8] . We currently lack a detailed knowledge of the specific molecular mechanisms underlying convergence at these phylogenetic depths. Butterfly wing patterns provide a unique opportunity to address the molecular basis of convergent evolution over deep evolutionary time because despite their incredible diversity, the wing patterns of this old evolutionary radiation are built from a conserved ground plan [9] . This permits us to investigate whether similar shifts in wing pattern among distantly related butterflies are controlled by homologous genes or pathways, and whether the causative nucleotide variation is conserved over evolutionary time [6] . Prior work suggests two very different predictions. On one hand, natural colour pattern variation routinely maps back to a core set of melanin pathway genes; this is true in both invertebrates [10] and vertebrates [11] , [12] , [13] , although the specific genes and pathways differ markedly between these two clades [14] . This suggests that the same pathway can be a recurrent target of selection for colour pattern variation in a given clade. In contrast, recent work on butterfly wing patterning suggests that its genetic basis is highly labile over evolutionary time. For instance, comparative analyses of gene expression show that while a set of developmental genes are used routinely for eyespot patterning [15] , [16] , [17] , the specific genes that are expressed in a given species and wing position are variable, as are the links between each gene and the adult phenotype it specifies. Furthermore, the gene optix has recently been shown to specify red and brown wing pattern elements in Heliconius butterflies, but not outside the genus, suggesting recent co-option in this one lineage [18] . Overall, these contrasting observations yield two very different hypotheses for the genetic control of butterfly wing pattern variation across deep evolutionary time, one predicting ancient homology and the other recent innovation. Positional cloning of the colour-patterning locus To investigate the genetic basis of wing pattern diversity, we first compared the genetic architecture of pattern formation in two butterfly systems, Limenitis and Heliconius , that exhibit convergent variation in mimetic colour patterns ( Fig. 1 ). Natural selection for mimicry between Limenitis and its unpalatable model, Battus philenor , has produced a hybrid zone between wing pattern races of Limenitis arthemis [19] , a non-mimetic, white-banded (ancestral) form and an unbanded, mimetic (derived) form. We used crosses between mimetic ( L. a. astyanax ) and non-mimetic ( L. a. arthemis ) individuals to map the position of the genomic region controlling mimetic wing pattern variation ( Supplementary Fig. 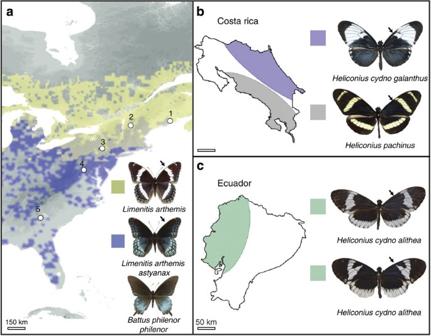Figure 1: Biogeographic distribution of study populations. (a) Parapatric distribution of hybridizing mimetic (L. a. astyanax)and non-mimetic (L. a. arthemis) admiral butterflies (distribution data from BAMONA59). White dots indicate population samples; note that the toxic model,B. philenor, geographically overlaps with the distribution of the mimetic form ofLimenitis60. (b) Parapatric distribution ofH. c. galanthusandH. pachinusin Costa Rica. (c) Sympatric distribution ofH. c. alitheain Ecuador. Black arrows illustrate medial pattern polymorphism on the forewing. Black arrows in each panel highlight variation in the melanic forewing pattern of each species. Scale bars in kilometres. 1 and Supplementary Table 1 ). Our crosses revealed that white-band patterning in Limenitis segregates as a single Mendelian locus, and based on syntenic comparisons maps to a homologous chromosomal position in Heliconius that is known to contain the colour-patterning locus, Ac ( Supplementary Fig. 1 ). Martin et al . [20] demonstrated that the Ac locus, which controls medial pattern shape in Heliconius forewings, maps to a genomic interval containing the diffusible signalling ligand WntA . WntA is a member of a larger family of Wnt signalling genes [21] that encode secreted ligands involved in cell signalling across a wide range of developmental processes [22] including examples of insect pigmentation [23] , [24] . By fine-mapping the colour-patterning chromosome in Limenitis , we reduced the zero-recombinant window to a 291-kb interval that contained just three genes, two chitin synthase genes and WntA ( Supplementary Fig. 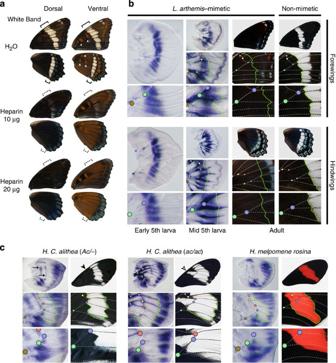Figure 2: Developmental expression ofWntAinLimenitisbutterflies. (a) Heparin or water injections of non-mimetic full-sibs at 8–16 h following pupation. Arrowheads indicate Discalis pattern elements known to express wingless61(syn.Wnt1). Heparin triggered a removal of the white band (bracket) and an expansion of the Discalis pattern elements (arrowheads), replicating previous results obtained inJunoniabutterflies29. (b) Developmental expression ofWntA in Limenitis5th instar larval wing discs. Vein intersections can be used as morphological landmarks for comparing the position of gene expression domains relative to the adult morphology (colour dots).WntAexpression delineates the proximal boundary of medial white bands (green line) from both banded and unbandedLimenitisstocks.WntAalso marks presumptive blue chevrons in the wing margin area during and after the mid-5th larval instar stage of wing development. (c) Spatial correspondence (green line) betweenWntAmRNA expression on larval wing discs and wing pattern contours among the polymorphicH. c. alitheamorphs species and in the sister speciesH. melpomene. Notice the presence of two stripes ofWntAexpression in the discal cell of (Ac/−) butterflies (arrows), correlating with theabsenceof a white element in this wing domain (arrowheads). TheAclocus was previously mapped to theWntAregion in this clade20. Asterisks indicate non-specific signal observed in tracheal tissues with thein situhybridization procedure. Scale bars, 1 cm (adult wings) and 500 μm (larval wings). 1 and Supplementary Table 2 ). Taken together, these results suggest that variation in the function or regulation of WntA likely mediates medial pattern formation in both Heliconius and Limenitis , two species that diverged 65 million years ago [25] . Figure 1: Biogeographic distribution of study populations. ( a ) Parapatric distribution of hybridizing mimetic ( L. a. astyanax) and non-mimetic ( L. a. arthemis ) admiral butterflies (distribution data from BAMONA [59] ). White dots indicate population samples; note that the toxic model, B. philenor , geographically overlaps with the distribution of the mimetic form of Limenitis [60] . ( b ) Parapatric distribution of H. c. galanthus and H. pachinus in Costa Rica. ( c ) Sympatric distribution of H. c. alithea in Ecuador. Black arrows illustrate medial pattern polymorphism on the forewing. Black arrows in each panel highlight variation in the melanic forewing pattern of each species. Scale bars in kilometres. Full size image Developmental patterns of gene expression To test this hypothesis, we examined the developmental basis of wing pattern formation in Limenitis using a combination of heparin injections, in situ hybridization ( Fig. 2 ) and RNA sequencing (RNAseq) experiments ( Fig. 3 ). First, to investigate WntA signalling, we injected heparin into early Limenitis pupae of a white-banded progeny. Heparin binds Wnt family ligands in a wide range of organisms, promoting their transport through the extracellular matrix of developing tissues [26] , [27] , [28] , and, in this case, resulted in a fully melanized adult wing pattern lacking the white band, similar to the mimetic form ( Fig. 2a ). These results, reminiscent of previous heparin injections in other butterfly species [20] , [29] , suggest a role for heparin-sensitive signals such as Wnt molecules in patterning the medial region of the butterfly wing. Next, we examined WntA expression in 5th larval instar wing discs and found that WntA mRNA expression forms an elongated antero-posterior expression domain ( Fig. 2b ) outside of the white band delineating the contour of its proximal boundary. This spatial correlation, observed in both forewings and hindwings, as well as across all observed stages ( Supplementary Fig. 2 ), suggests that WntA has a role in the early developmental specification of the white band. Despite this, we found identical spatial patterns of WntA expression in both the mimetic and the non-mimetic forms ( Fig. 2b and Supplementary Fig. 2 ). This result was surprising because spatial modulation of WntA mRNA expression is directly perceptible in the larval wing discs of Heliconius , and larval WntA expression domains perfectly mirror patterns of phenotypic variation on the adult wing ( Fig. 2c ; ref. 20 ). Therefore, to investigate whether an alternative mechanism operates in Limenitis , we then performed RNAseq analysis of WntA expression across four developmental time points (5th instar, prepupal, <48 post pupation and >48 post pupation), and found highly significant evidence for upregulated expression of a 5′-untranslated region (UTR), during the 5th instar stage, only among mimetic individuals ( Fig. 3 ; general linear model (GLM): n =6, P <0.0001 after false discovery rate (FDR) correction [30] ). Consistent with our in situ hybridization results, we also found that no other WntA exons were differentially expressed in Limenitis at any developmental time point examined. Figure 2: Developmental expression of WntA in Limenitis butterflies. ( a ) Heparin or water injections of non-mimetic full-sibs at 8–16 h following pupation. Arrowheads indicate Discalis pattern elements known to express wingless [61] (syn. Wnt1 ). Heparin triggered a removal of the white band (bracket) and an expansion of the Discalis pattern elements (arrowheads), replicating previous results obtained in Junonia butterflies [29] . ( b ) Developmental expression of WntA in Limenitis 5th instar larval wing discs. Vein intersections can be used as morphological landmarks for comparing the position of gene expression domains relative to the adult morphology (colour dots). WntA expression delineates the proximal boundary of medial white bands (green line) from both banded and unbanded Limenitis stocks. WntA also marks presumptive blue chevrons in the wing margin area during and after the mid-5th larval instar stage of wing development. ( c ) Spatial correspondence (green line) between WntA mRNA expression on larval wing discs and wing pattern contours among the polymorphic H. c. alithea morphs species and in the sister species H. melpomene . Notice the presence of two stripes of WntA expression in the discal cell of ( Ac/− ) butterflies (arrows), correlating with the absence of a white element in this wing domain (arrowheads). The Ac locus was previously mapped to the WntA region in this clade [20] . Asterisks indicate non-specific signal observed in tracheal tissues with the in situ hybridization procedure. Scale bars, 1 cm (adult wings) and 500 μm (larval wings). 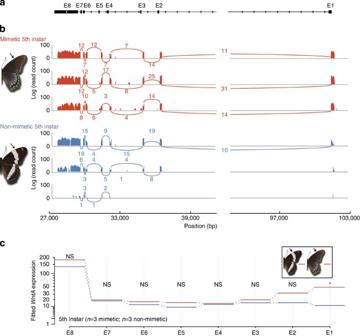Figure 3: Differential expression of 5′-UTR ofWntAin 5th InstarLimenitisbutterflies. (a) Exon and intron structure of theWntAgene is shown. The 5′ end of theWntAgene is shown on the right, and the direction of translation predicted is shown. E8 denotes the 5′-UTR E2–E8 represent the coding exons of theWntAgene. (b) Log-scaled RNAseq read counts for three mimetic (red) and three non-mimetic individuals (blue) are shown. Number of reads spanning exons are indicated with curved lines. (c) Using the software package DEXSeq30, we modelled exon expression between mimetic and non-mimetic individuals using a general linear model (GLM). GLM fitted expression values for each mimetic and non-mimetic individual are shown for each exon. No statistical difference was observed for exons E2–E8, however, we detected significant (GLM:n=6,P<0.0001) differential exon usage of the 5′-UTR (E1) between mimetic (n=3) and non-mimetic (n=3)Limenitisonly during the 5th instar stage. NS, not significant. Arrows indicate presence and absence of white band in mimetic and non-mimetic Limenitis respectively. Asterisk indicates significant differential expression (P<0.0001). Full size image Figure 3: Differential expression of 5′-UTR of WntA in 5th Instar Limenitis butterflies. ( a ) Exon and intron structure of the WntA gene is shown. The 5′ end of the WntA gene is shown on the right, and the direction of translation predicted is shown. E8 denotes the 5′-UTR E2–E8 represent the coding exons of the WntA gene. ( b ) Log-scaled RNAseq read counts for three mimetic (red) and three non-mimetic individuals (blue) are shown. Number of reads spanning exons are indicated with curved lines. ( c ) Using the software package DEXSeq [30] , we modelled exon expression between mimetic and non-mimetic individuals using a general linear model (GLM). GLM fitted expression values for each mimetic and non-mimetic individual are shown for each exon. No statistical difference was observed for exons E2–E8, however, we detected significant (GLM: n =6, P <0.0001) differential exon usage of the 5′-UTR (E1) between mimetic ( n =3) and non-mimetic ( n =3) Limenitis only during the 5th instar stage. NS, not significant. Arrows indicate presence and absence of white band in mimetic and non-mimetic Limenitis respectively. Asterisk indicates significant differential expression ( P <0.0001). Full size image Population genomics Next, to characterize patterns of nucleotide variation across the colour-patterning region in Limenitis , we generated a single, contiguous reference scaffold by sequencing bacterial artificial chromosome (BAC) clones spanning our zero-recombinant interval ( Fig. 4a ). Subsequent sequencing and analysis of 30 full Limenitis genomes ( Supplementary Table 2 ), including both parents of the mapping brood, aligned to our BAC reference, identified a 30-kb segregating haplotype, consisting of 173 fixed single-nucleotide polymorphisms (SNPs) in complete linkage disequilibrium (LD), located 23 kb upstream of the 5′ coding region of WntA , which predicts phenotype across all samples ( Fig. 4b and Supplementary Fig. 3 ). To verify this result, we genotyped an additional 120 butterflies across a transect of the phenotypic hybrid zone between these two wing pattern races, and, again, found a perfect correspondence between genotype and phenotype ( Fig. 5 ; Supplementary Fig. 3 and Supplementary Table 2 ). Importantly, genome-wide patterns of molecular variation revealed no evidence of geographic population structure [19] ( Supplementary Figs 5 and 6 ; and Supplementary Tables 3 and 4 ), and no other portion of the genome showed an association with phenotype. In addition, because we found no overlap between associated SNPs and the WntA exons, these results rule out coding mutations as a possible molecular switch controlling the presence/absence of white bands in Limenitis . Finally, to investigate the mechanism maintaining extended LD upstream of WntA , we analysed patterns of structural variation, and found evidence for a single 9-kb-long interspersed element (LINE) retrotransposon, situated near the centre of the mimetic haplotype but absent in the non-mimetic allele, that occurs in the 60-kb-long first intron of WntA that was also perfectly associated with phenotype ( Fig. 3b , vertical blue bar, and Supplementary Fig. 4 ). LINE elements can suppress recombination via the insertion of a non-homologous and non-collinear sequences, as well as by altering local DNA methylation patterns [31] , and, therefore, may be responsible for maintaining LD across the large (30 kb) haplotypes we found. 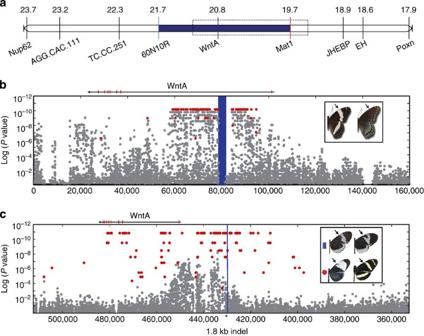Figure 4: SNP associations with mimetic polymorphisms withinLimenitisandHeliconius. (a) The zero-recombinant colour-patterning interval inLimenitis(blue). (b) Variable SNPs (grey) mapped by position (xaxis) against thePvalue for the Fisher’s exact test of allelic association with phenotype (yaxis); SNPs fixed between mimetic and non-mimeticLimenitisindividuals are shown in red. The highlighted blue interval corresponds to the position of a long interspersed element (LINE) retrotransposon fixed between mimetic and non-mimetic individuals. (c) SNPs mapped across the chromosome containingWntAinH. c. alithea(grey), with position on thexaxis, andPvalue of Fisher’s exact test for allelic association on theyaxis for the melanic/non-melanic phenotypes. There were no fixed SNPs between these two phenotypes; however, 170 fixed differences were detected among comparisons of allopatricH. c. galanthusandH. pachinus(red). Combined analysis of structural variation inH. c. alitheaand all otherHeliconiusstudies revealed a single 1.8-kb indel that was perfectly associated with variation in forewing melanin patterning (black arrows), which is positionally highlighted in blue for all species sequenced. Figure 4: SNP associations with mimetic polymorphisms within Limenitis and Heliconius. ( a ) The zero-recombinant colour-patterning interval in Limenitis (blue). ( b ) Variable SNPs (grey) mapped by position ( x axis) against the P value for the Fisher’s exact test of allelic association with phenotype ( y axis); SNPs fixed between mimetic and non-mimetic Limenitis individuals are shown in red. The highlighted blue interval corresponds to the position of a long interspersed element (LINE) retrotransposon fixed between mimetic and non-mimetic individuals. ( c ) SNPs mapped across the chromosome containing WntA in H. c. alithea (grey), with position on the x axis, and P value of Fisher’s exact test for allelic association on the y axis for the melanic/non-melanic phenotypes. There were no fixed SNPs between these two phenotypes; however, 170 fixed differences were detected among comparisons of allopatric H. c. galanthus and H. pachinus (red). Combined analysis of structural variation in H. c. alithea and all other Heliconius studies revealed a single 1.8-kb indel that was perfectly associated with variation in forewing melanin patterning (black arrows), which is positionally highlighted in blue for all species sequenced. 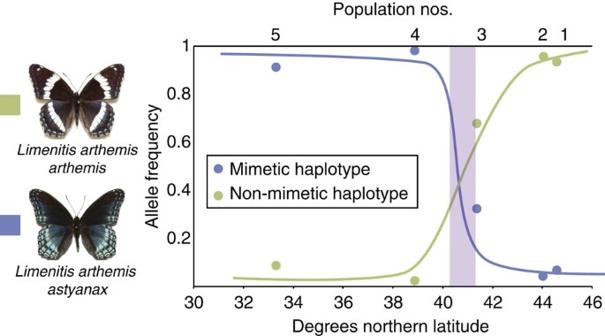Figure 5: Allele frequencies ofWntAhaplotypes across the phenotypic hybrid zone between mimetic and non-mimetic populations ofLimenitis. Population numbers correspond to sampling localities. The light purple shading indicates the geographic position of the hybrid zone. Full size image Figure 5: Allele frequencies of WntA haplotypes across the phenotypic hybrid zone between mimetic and non-mimetic populations of Limenitis . Population numbers correspond to sampling localities. The light purple shading indicates the geographic position of the hybrid zone. Full size image Taken together, our results suggest that differential expression of a WntA 5′-UTR sequence during late larval development underlies adaptive phenotypic divergence between mimetic and non-mimetic Limenitis . At the molecular level, differential expression of the 5′-UTR may have arisen either directly (by interfering with gene function) or indirectly (by facilitating the accumulation of cis-regulatory mutations) from a LINE insertion in the first intron of WntA . Alternatively, the extensive LD we observed may instead reflect strong natural selection on multiple cis-regulatory SNPs interspersed across the haplotype interval. Under either scenario, differential expression of the 5′-UTR is a reasonable proximate mechanism given that such sequences regulate many aspects of protein translation [32] , and, in this case, the differentially expressed WntA 5′-UTR contains a predicted internal ribosome entry site (IRES) motif that could mediate such effects ( Supplementary Fig. 7 ). This latter observation suggests that a post-transcriptional regulatory mechanism may act as the molecular switch in Limenitis , controlling the presence/absence of white bands. Comparative genomics of colour pattern evolution While these results provide unique insights into the molecular basis of adaptation, our primary goal was to identify and compare the proximate basis of melanin pattern formation in Limenitis and Heliconius . To do this, we first focused on two closely related species in Costa Rica, H. cydno galanthus ( n =10) and H. pachinus ( n =10), which vary markedly in their Müllerian mimicry phenotypes as a result of allelic variation at Ac [20] ( Fig. 4c ); H. pachinus has a melanized patch of scales, which is lacking in H. c. galanthus . Examination of SNPs across the 581-kb Ac scaffold from the published Heliconius genome sequence [33] identified 170 SNPs and a 1.8-kb indel fixed between these two species, all of which occur upstream of the WntA coding region. To refine the phenotypic association, we then analysed an additional 25 genomes from a single phenotypically variable population of H. c. alithea in Ecuador, in which similar Ac phenotypes segregate as a polymorphism [34] ( Fig. 4c ). This analysis ruled out all SNPs and revealed a single structural variant, the 1.8-kb indel, that is perfectly associated with forewing pattern shape in Heliconius from Costa Rica and Ecuador ( Supplementary Fig. 8 ). In fact, the Ac locus was previously mapped to WntA in laboratory crosses, and pure-bred stocks of each Ecuadorian morph show discrete differences in WntA expression that explain their pattern differences ( Fig. 2c ). Collectively, these results strongly suggest that structural variation upstream of WntA contributes directly to cis -regulatory divergence among morphs of H. c. alithea . Finally, alignment of the WntA interval from Heliconius and Limenitis ( Fig. 4b,c ) revealed that the mutational variants overlap in both systems, supporting the hypothesis that phenotypic convergence originated as a consequence of cis -regulatory mutations influencing developmental patterns of gene expression in the same gene, WntA . Convergent phenotypic evolution among distinct evolutionary lineages is generally considered evidence for adaptation, thereby illustrating the power of natural selection to shape patterns of morphological evolution [35] . In contrast, convergence at the molecular level is often viewed as a consequence of generative constraints, with certain genetic or developmental architectures limiting the functional mechanisms available in the production of novel morphologies [35] , [36] . With the maturation of the genomic age comes the ability to examine the molecular basis of phenotypic evolution at multiple functional levels [13] , [37] and in multiple biological systems. Such work promises to reveal the extent to which the evolutionary process is predictable over varying evolutionary timescales [36] , [38] , [39] . While several studies have identified instances of genetic parallelism over large divergence times ( Fig. 6 and Supplementary Data 1–3 ), we note that ascertainment biases on genetic function may favour the discovery of genetic parallelism in studies that repeatedly focus on the same small sets of candidate genes. 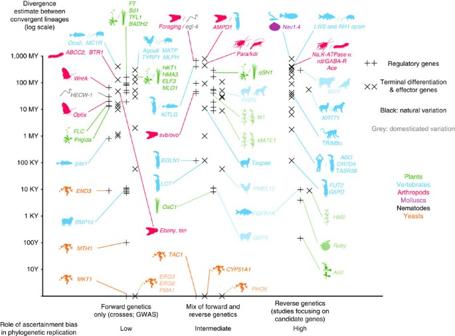Figure 6: The empirical landscape of parallel genetic evolution. The graph features 118 genes involved in parallel genetic evolution, wherede novomutations have independently driven phenotypic evolution of a phenotypic trait in at least two lineages. Theyaxis marks the estimated divergence time between the two lineages (for genes with >2 entries, the most distant pair is shown). The literature is also partitioned across thexaxis according to criteria thought to influence the discovery of parallel genetic evolution: (1) type of ascertainment bias on the genetic nature of the trait38; (2) cases of natural variation versus cases including domesticated variation38; and (3) regulatory versus terminal differentiation and effector genes39. SeeSupplementary Data 1–3for data and references. Figure 6: The empirical landscape of parallel genetic evolution. The graph features 118 genes involved in parallel genetic evolution, where de novo mutations have independently driven phenotypic evolution of a phenotypic trait in at least two lineages. The y axis marks the estimated divergence time between the two lineages (for genes with >2 entries, the most distant pair is shown). The literature is also partitioned across the x axis according to criteria thought to influence the discovery of parallel genetic evolution: (1) type of ascertainment bias on the genetic nature of the trait [38] ; (2) cases of natural variation versus cases including domesticated variation [38] ; and (3) regulatory versus terminal differentiation and effector genes [39] . See Supplementary Data 1–3 for data and references. Full size image Here we have leveraged the power of association mapping in naturally hybridizing populations to demonstrate that a positionally orthologous region of the WntA locus has independently driven the evolution of mimetic wing patterns in two butterfly species. Although additional functional work is needed to evaluate the regulatory consequences of these mutations, the discovery of parallel genetic evolution of WntA is remarkable (1) because it was identified in two independent mapping studies without initial bias on the genetic basis of the trait (2) owing to the exceptionally large divergence times ( ca . 65 MY) between Heliconius and Limenitis , and (3) because, unlike melanin pathway genes that have also been repeatedly linked to pigment variation, WntA is a regulatory gene involved in the early deployment of spatial information in undifferentiated tissues (for example, embryos [40] and wing discs). Surprisingly, our results suggest that modulation of this conserved developmental gene has occurred in tandem between these two deeply divergent butterfly lineages, implying an unexpected and remarkable level of predictability in the evolutionary process. Positional cloning All Limenitis specimens utilized for genetic linkage mapping were collected from a single locality in Pennsylvania ( Supplementary Table 2 ). Wild-captured, mated female specimens were captured and fed a mixture of honey and water twice daily, and were secured on Prunus serotina and/or Salyx babylonica to encourage oviposition. Larvae were raised directly on host plants with one brood per enclosure. Pupae were collected and placed in labelled containers to prevent adults from mating upon emergence. Adult butterflies were transferred to envelopes numbered with their sibling group and according to their order of emergence. Adults were then photographed and crossed via hand-pairing [41] . Mapping families were generated via backcrossing heterozygous mimetic males to fully banded, non-mimetic females (homozygous recessive at the major gene controlling mimicry), as linkage maps constructed with heterozygous females are uninformative because there is no recombination during oogenesis [42] . Following mating, the wings and tissues of male butterflies were immediately archived, and the wings and tissues of female butterflies were archived when oviposition was ceased. Progeny from mapping crosses were photographed upon emergence, and wings and tissues were archived. Medial banding in Limenitis is controlled by two, incompletely dominant, alleles at a single locus [43] , and at least one dominant modifier that influences the penetrance of the white-banded allele in heterozygous individuals. All progeny from mapping crosses displayed either the mimetic phenotype (heterozygous with dominant modifier) or the white-banded (homozygous) phenotype. We scored wing patterns of the resulting 111 progeny of the mapping family based on the presence or absence of hindwing and forewing medial white banding. Forty-five were mimetic (23 males and 22 females) and 66 were fully banded (30 males and 36 females; χ 2 =3.973, two-tailed P value=0.046). Although these values differ weakly from our statistical expectations, the results of numerous other crosses carried out by SPM over the last 10 years support a model of Mendelian inheritance. Wings were removed from each butterfly, photographed and archived in glassine envelopes. Remaining whole bodies were placed inside 1.5 ml microcentrifuge tubes with 100% ethanol to preserve the genomic DNA. Wing muscle tissue was dissected from each archived butterflies, and DNA extractions were performed using the DNeasy Blood and Tissue Kit (Qiagen, Inc.). Amplified fragment length polymorphism (AFLP) genotypes were generated using the AFLP Plant Mapping kit for small plant genomes (Applied Biosystems, Inc.) following the manufacturer’s instructions. In brief, fragments were generated using restriction enzymes EcoRI and MseI. Next, fragments were ligated to adaptors and selectively amplified during two separate rounds of PCR. Once the PCRs was completed, reactions for each fragment were spiked with an internal lane size standard to ensure proper size matching of AFLP across samples. Fragment analysis was performed on an 3730xl DNA Analyzer (Applied BioSystems, Inc.). AFLP electropherograms were analysed in Applied Biosystem’s GeneMapper software, version 3.7 (Applied Biosystems, Inc.), with AFLP alleles scored as either present or absent and according to fragment size. Peak height threshold was set to 80 RFU. Fragments smaller than 50 base pairs and larger than 550 base pairs were excluded from analysis. The parents and progeny ( n =111) were then genotyped for 60 unique AFLP primer pair combinations [44] analysed separately in GeneMapper, version 3.7 (Applied Biosystems, Inc.), and any marker that had a large number of missing genotypes was removed from the data set. Of the resulting 2,571 AFLP, 506 (19.7%) were diagnostic, mappable markers (present in the male, absent in the female and segregating in the progeny in a near 1:1 pattern). AFLP marker order and position were estimated using JoinMap 3.0 (ref. 45 ), which used χ 2 -tests for segregation distortion and tests of independence to filter spurious genotypes. Log likelihood ratio scores above 3.0 for markers are considered significant evidence for linkage (95% probability). Markers were separated into linkage groups and are selected for mapping at a minimum log likelihood ratio score of 4.0. Final map distances were corrected using Kosambi’s mapping function; this function is designed to account for the observation that larger chromosomes are more likely to have double crossovers than small chromosomes and results in shorter, more accurate linkage maps compared with those maps using Haldane’s mapping function that assumes complete interference [45] . Mapping of the diagnostic markers resulted in 30 linkage groups, varying in length from 46 to 107 cM, and in agreement with chromosomal number estimates for this species [46] . The total map length was 2,250 cM with an average distance of 4.5 cM between AFLP markers. Given the genome size estimate for Limenitis [47] of 388 Mb (+/− 7 Mb for females and 4 Mb for males), each cM in our map represents ~160.4 kb. Direct comparisons among linkage maps based on dominant markers, such as AFLPs, are not possible. Therefore, we generated diagnostic SNP markers from highly conserved nuclear genes by designing Limenitis -specific primers from annotated expressed sequence tags (ESTs) developed via 454 pyrosequencing of 48 h pupal wing disc cDNA, and genotyped the entire backcross mapping brood for each SNP by Sanger sequencing to facilitate comparisons with other published Lepidopteran genetic maps, with an emphasis on Heliconius . Such comparisons are greatly facilitated in Lepidoptera because macrosynteny is highly conserved [33] , [48] , [49] , thereby allowing direct identification of homologous chromosomal linkage groups across systems. The final linkage map contains 57 SNPs from 54 conserved nuclear genes, such as 506 AFLPs, 1 BAC end sequence and 2 colour pattern loci ( wbd and ird ), providing 565 distinct markers with a total map distance of 2,248 cM across 30 linkage groups (only the W chromosome was not mapped). The average linkage group was 74.9 cM. Both the total map length and the average linkage group length remained nearly the identical to the dominant marker map. However, the addition of 57 new SNPs reduced the average distance between markers from 4.44 to 3.99 cM, an estimated 6,000 bp difference per cM. Importantly, mapping of the nuclear genes demonstrated that mimetic variation in Limenitis segregates with several genes known to be linked to the chromosome in Heliconius , which is known to house the colour-patterning locus, Ac [50] . The addition of 19 syntenic nuclear markers [49] known to be linked to Ac in Heliconius ( Supplementary Fig. 1 and Supplementary Table 1 ) resulted in a more accurate positioning of markers on the Limenitis wing patterning chromosome, and reduced the zero-recombinant mapping interval to a 2-cM region containing two adjacent chitin synthase genes and the candidate gene, WntA [20] . Developmental patterns of gene expression and functional tests Mimetic and non-mimetic female Limenitis were wild captured from Baltimore county, Maryland, and White Mountain National Forest, New Hampshire, respectively. Lab-reared offspring from true-breeding individuals were mated to full-sibs, and the resulting progeny were utilized as reported for all following developmental and functional tests. Pupae aged 8–16 h after pupation were injected with 10 or 20 μg μl −1 heparin or sterile H 2 O using a pulled glass micropipette mounted on a 10-μl cut pipette tip and a 2–20- μl pipette. Pupae were surface sterilized with ethanol and injected on the left side in an interstice that separates the baso-posterior parts of the developing forewing and hindwing. As in previous reports [20] , H 2 O controls showed no effects, heparin had systemic effects on both left and right wing patterns, and control and heparin injections did not produce local damage artefacts. All of the results presented in Fig. 2 were replicated at least three times per morph and dosage (including H 2 O control). Individual mimetic and non-mimetic Limenitis were sampled at the 5th instar stage of development ( Supplementary Fig. 2A ). Each individual was anaesthetized in ice-cold water and their wing discs dissected in PBS, incubated in cold fixative (formaldehyde 9% in PBS containing 50 mM EGTA) for 30–35 min, rinsed in PBS with 0.01% Tween20 (PBST), and then dehydrated with increasing concentrations of methanol and kept for long-term storage in methanol at −20 °C. For in situ hybridization, we followed the method described in ref. 20 . In brief, wing discs preserved in methanol were rehydrated in increasing concentrations of cold PBST, washed in cold PBST and freed from their peripodial membrane using fine forceps. The tissues were then post fixed 20 min on ice in PBS containing 5.5% formaldehyde, transferred to a standard hybridization buffer, incubated in supplemented hybridization buffer for 16–40 h at 62 °C. Tissues were washed eight times, and, then for secondary detection of the riboprobe, the tissues were blocked and then incubated with a 1:4,000 dilution of anti-digoxigenin alkaline phosphatase Fab fragments (Roche Applied Science, Indianapolis, Indiana, USA). Tissues were again washed 10 times for 10–120 min, and finally stained with BM Purple (Roche Applied Science) for 4–8 h at room temperature. Stained tissues were then washed in PBST 2 mM EDTA and slide mounted in PBS containing 60% glycerol. mRNA in situ hybridizations were photographed with a Nikon Coolpix P5100 digital camera (Nikon Inc., Melville, New York, USA) mounted with a LNS- 30D/P51 adapter (Zarf Enterprises, Spokane, Washington, USA) on a Leica S4E microscope (Leica Microsystems, Buffalo Grove, Illinois, USA). Mimetic and non-mimetic individuals were captured in Massachusetts and New Hampshire, respectively, and allowed to oviposit in the laboratory. Mimetic and non-mimetic individuals were then crossed to siblings to ensure that they were true-breeding for each respective phenotype. Individuals from each cross were sampled at the 5th instar ( n =3 mimetic and n =3 non-mimetic), prepupa (identified by stereotypic ‘j-curve’ hanging from leaves; n =3 mimetic and n =3 non-mimetic), early pupation (<48 h post pupation; n =3 mimetic and n =3 non-mimetic), and late pupation (>48 h post pupation; n =3 mimetic and n =3 non-mimetic). Wing discs were dissected from each individual in cold PBS, wing discs were then stored in RNAlater (Ambion, Inc.) following manufacturer’s instructions. RNA was extracted using an RNAeasy-kit (Qiagen, Inc.), and individual RNAseq libraries were prepared using the TrueSeq RNA sample prep kit (Illumina, Inc.) at the Michigan State University Genomics core facility. Each library pooled, and pools were sequenced across two lanes of an Illumina HiSeq 2500, using 2 × 150 bp reads. Individual reads were quality filtered and trimmed using custom python scripts, then aligned to BAC sequences representing mimetic and non-mimetic haplotypes using the TopHat pipeline [51] . TopHat identified genes and exons automatically based on read alignment. Differential expression of whole genes was determined using Cufflinks [51] , and differential expression of exons was determined using DEXSeq [30] . Differential expression of the WntA was not detected at any developmental stage. Differential expression of WntA exon 1 was detected between mimetic and non-mimetic individuals only in the 5th instar stage, where WntA expression is highest ( P <0.0001 after Benjamini–Hochberg correction for false positives). Generation of BAC tile path A custom Limenitis BAC library was constructed from eight individuals captured from a single hybrid population from Pennsylvania ( Supplementary Table 1 ). Nylon arrays of BAC clones were prepared by Amplicon Express (Pullman, WA), and were screened using Mat1 and WntA probes. Of the entire library of ~18,000 clones, 10 BACs screened positive for Mat1 , 9 BACs screened positive for WntA and 1 clone, 21G6, screened positive for both markers. These 19 clones were selected for end sequencing and high-depth next-generation Illumina sequencing and assembly, performed by Amplicon Express. Because of considerable structural variation between these BAC contigs, sequences were aligned in multiple steps. First, BAC end sequences of all 19 clones were mapped using BLAST to each individual contig, and clones were aligned manually. Next, when a tile of multiple contigs spanning the zero-recombinant interval was determined, we performed a final alignment of the constituent BAC contigs using the MAFFT [52] algorithm as implemented by Genious Pro (Biomatters, Inc.). The final reference was comprised of three major contigs representing clones from 21G6, 60N10 and 70O17. A fourth BAC contig, 43D10, contained the alternative Limenitis haplotype reported in the text. The assembled reference sequence for the zero-recombinant interval (‘ Limenitis AC scaffold’) used for our comparisons contained the haplotype typical of the mimetic, unbanded phenotype. A FASTA file containing all BAC sequences is available as a supplementary file ( Supplementary Data 4 ). Population genomic resequencing We collected adult butterflies for DNA sampling from a variety of locations ( Supplementary Table 1 ), representing 120 individual Limenitis spp from sites in Georgia, Virginia, Vermont, Pennsylvania and Maine, as well as 25 H. c. alithea from sites in Ecuador, and finally 10 additional localities in Costa Rica, representing H. c. galanthus ( n =10) and H. pachinus ( n =10). All samples were euthanized, and then wings were separated and placed in glassine envelopes while the bodies were stored in 95% ethanol. For each sample, we extracted DNA from butterfly wing muscles using DNAeasy kits (Qiagen, Inc.) following manufacturer’s instructions. For Limenitis and H. c. alithea , we performed short-read genomic library construction using the Nextera Sample Preparation kit, following the manufacturer’s instructions. These libraries were sequenced using an Illumina HiSeq 2000, with 2 × 150 bp paired-end reads, at the Bauer Sequencing Core Facility (Harvard University) to ~10 × coverage per individual. We subsequently generated ~8 × coverage for both parents of our backcross mapping brood using 2 × 250 bp MiSeq runs. For the remaining Heliconius spp., a custom Illumina sequencing library with a 500-bp insert was prepared for each sample and sequenced to an average depth of 16 × coverage using an Illumina HiSeq 2000 (2 × 100 paired-end sequencing). Library preparation and sequencing were performed at the Beijing Genome Institute. This sequencing data is archived in the NCBI Short Read Archive with the following BioProject accession number: PRJNA226620 . All remaining Limenitis and H. c. sequencing data is archived in the NCBI Short Read Archive with the following accession BioProject accession number: PRJNA252628 . BAC sequence alignment Limenitis spp : Following sequencing, sequence libraries representing each sample were trimmed and filtered for quality using the fastx toolkit (CSHL), scythe and sickle (UC-Davis). Next, filtered reads were aligned to the Limenitis reference BAC tile path (see the section ‘Generation of BAC tile path’) using the ‘very fast’ parameter set with local alignment. SNPs were called simultaneously for all samples using the multi-allelic calling function in GATK version 1.5 (refs 53 , 54 ). Positions with a total SNP quality <40 were filtered from subsequent analyses. This resulted in a data set containing 9896 SNPs. A custom perl pipeline was used to identify biallelic SNPs within this data set that were fixed between phenotypes. Average pairwise LD, for SNPs was calculated as the squared correlation coefficient ( r 2 ) between allele counts observed between each SNP and its 200 nearest neighbours (5,000 bp, maximum distance) using the VCFtools software package [55] . Average r 2 at this location was then was then calculated for all r 2 values, and the process was repeated. This approach is computationally feasible for large data sets since it does not require haplotype reconstruction, but it provides only an approximation of the true LD [56] . Based on these analyses, we identified a large (30 kb) segregating haplotype that was perfectly association with wing pattern phenotypes in Limenitis ( Supplementary Fig. 3 ). Hybrid zone transect genotyping To further investigate the phenotypic association between Limenitis wing pattern morphs and the segregating haplotype, we designed a TaqMan probe-based gene expression assay using custom primers. The two probes, which were haplotype specific, were labelled with a FAM or VIC dye label on the 5′ end, and a minor grove binder non-fluorescent quencher on the 3′ end. We PCR amplified all individuals using a 20-μl volume, following the manufacturer’s suggested conditions, and then took end point fluorescence measurements, using an Eppendorf RealPlex2 mastercycler, to call heterozygotes and both homozygote genotypes. The frequency of each haplotype relative to geographic sampling locality is shown in Fig. 4 . The presence of heterozygous individuals in populations outside of the hybrid zone reflects geographic differences in the frequency of alleles at the modifying locus. Previous crossing experiments indicate that the dominant modifier is at high frequency near the hybrid zone but declines in frequency with increasing geographic distance from the hybrid zone. Population structure tests To test the null hypothesis of geographic population structure, non-mimetic ( L. a. arthemis ) and mimetic ( L. a. astyanax ) butterflies ( n =417 individuals) were sampled across two independent transects of the hybrid zone ( n =10 populations/transect; Supplementary Table 3 ), and genotyped with 12 selective AFLP primer combinations following the same protocol described above (see Genotyping). The 12 unique AFLP primer pair combinations resulted in the presence or absence of 2,723 AFLP loci, of which 490 AFLPs had a minor allele frequency ≥0.10 and were retained for subsequent analyses ( Supplementary Table 4 ). Outlier analysis was then performed to identify loci experiencing selection using the programme BAYESCAN v. 2.0 (ref. 57 ). Within BAYESCAN, estimation of model parameters was tuned automatically on the basis of short pilot runs (10 pilot runs, length 5,000), using default chain parameters. Loci were then ranked according to their estimated posterior probability, and all loci showing log(Bayes Factor)>2 ((P[ai] 6¼ 0)>0.99) were treated as outliers ( Supplementary Fig. 5 ). Partitioning the AFLP data into outlier ( n =62; FDR=0.001) and non-outlier ( n =428) loci revealed low overall population differentiation (F ST neutral=0.09 versus 0.51 for outliers) and no evidence for population structure based on wing pattern. We also used the programme STRUCTURE v. 2.2 (ref. 58 ) to cluster individuals from each transect on the basis of their multilocus AFLP genotypes. For both transects, clustering runs (burn-in=5,000 repetitions and main run=5,000,000 repetitions) using the admixture model, and allowing the number of clusters to vary from K =1 to 10, returned the maximum log likelihood value for K =4. However, inspection of the clustering results indicates no correspondence between individual genotypes and geography or wing pattern ( Supplementary Fig. 6 ). Ac reference sequence alignment H. c. alithea : The described procedure for Limenitis was followed, except sequences were aligned to the H. melpomene scaffold known to contain the WntA gene [20] . The NCBI GenBank accession number for this scaffold is HE668478 . This resulted in a data set containing 37,347 SNPs. Additional Heliconius species : Reads were trimmed and filtered for quality as described above. These additional Heliconius species were subsequently aligned to the Hmel 1.1 reference genome [33] using Stampy [55] . SNPs were called simultaneously for all Heliconius spp samples using the multi-allelic calling function in GATK version 1.5 (refs 53 , 54 ). Positions with a total SNP quality <40 were filtered from subsequent analyses. This resulted in a data set containing 42,522 SNPs. We found a single 1.8-kb indel that was perfectly associated with allelic variation in Ac phenotypes among H. c. galanthus , H. pachinus and the two phenotypes of H. c. alithea ( Supplementary Fig. 8 ). How to cite this article: Gallant, J. R. et al . Ancient homology underlies adaptive mimetic diversity across butterflies. Nat. Commun. 5:4817 doi: 10.1038/ncomms5817 (2014). Accession codes: All Illumina short reads have been archived in the NCBI Short Read Archive with the following BioProject accession numbers: PRJNA226620 and PRJNA252628 .